Self-assembled aggregates formed by single-molecule magnets on a gold surface The spontaneous ordering of molecules into two-dimensional self-assembled arrays is commonly stabilized by directional intermolecular interactions that may be promoted by the addition of specific chemical side groups to a molecule. In this paper, we show that self-assembly may also be driven by anisotropic interactions that arise from the three-dimensional shape of a complex molecule. We study the molecule Mn 12 O 12 (O 2 CCH 3 ) 16 (H 2 O) 4 (Mn 12 (acetate) 16 ), which is transferred from solution onto a Au(111) substrate held in ultrahigh vacuum using electrospray deposition (UHV-ESD). The deposited Mn 12 (acetate) 16 molecules form filamentary aggregates because of the anisotropic nature of the molecule–molecule and molecule–substrate interactions, as confirmed by molecular dynamics calculations. The fragile Mn 12 O 12 core of the Mn 12 (acetate) 16 molecule is compatible with the UHV-ESD process, which we demonstrate using near-edge X-ray adsorption fine-structure spectroscopy. UHV-ESD of Mn 12 (acetate) 16 onto a surface that has been prepatterned with a hydrogen-bonded supramolecular network provides additional control of lateral organization. The bottom-up self-assembly of two-dimensional arrays of molecules and nanoparticles with inherent optical, chemical, tructural and magnetic functionalities requires a detailed understanding and control of intermolecular forces [1] , [2] , [3] , [4] , [5] , [6] , [7] , [8] , [9] . In much of the work in this area, highly directional interactions, such as hydrogen bonding or metal coordination, are exploited to promote the formation of arrays with controlled structural characteristics. There has been great success in this approach, particularly when applied to relatively simple molecules or particles with high symmetry. For larger, more complex moieties, the influence of intermolecular interactions is much more difficult to predict, as anisotropies result from a balance between the three-dimensional shape of a molecule or nanoparticle and its surface chemistry. In this paper, we describe the structures that emerge when the molecule Mn 12 (acetate) 16 is deposited on a metallic surface under vacuum. The molecule Mn 12 (acetate) 16 provides an interesting and well-studied example of a large, complex molecule and has attracted considerable interest because of its intrinsic magnetic functionality. Mn 12 (acetate) 16 molecules are potential candidates for high-density magnetic memory devices because of their bistability [10] , and models have been proposed for their use within the field of quantum computation [11] . Of particular relevance to this paper is the complex three-dimensional molecular shape that leads directly to the spontaneous formation of filamentary structures through the aggregation of diffusing Mn 12 (acetate) 16 . In this context, Mn 12 (acetate) 16 provides an exemplar of a nanoscale object with a complex intermolecular potential in which anisotropies arise from the asymmetric shape of the molecule rather than through interactions that are intrinsically anisotropic. Accordingly, our results are expected to have wide relevance to the surface self-assembly of other large molecules, as well as direct relevance to lateral ordering of Mn 12 (acetate) 16 for technological applications. The molecule investigated here is based on the mixed valence dodecamanganese cluster, which contains four Mn 4+ ions within the core and eight Mn 3+ ions around the periphery. The magnetic core is protected by an organic shell that may be altered by conventional wet chemistry techniques such as ligand exchange [12] , [13] , [14] and direct synthesis from the appropriate carboxylate reagents [15] . Mn 12 (acetate) 16 exhibits magnetic properties, such as hysteresis cycles, magnetic anisotropy originating from a purely molecular basis [10] , [16] , quantum magnetic tunnelling effects [17] , [18] and also has potential for molecular information storage devices [11] , [19] . Lateral organization is highly relevant to all these applications, although so far there have been relatively few high-resolution studies to determine the influence of intermolecular interactions on the packing and ordering of molecules. This is partly because of the fragile nature of Mn 12 (acetate) 16 , which makes them unsuitable for sublimation and largely precludes the investigation of derived thin films using high-resolution techniques such as ultrahigh vacuum (UHV) scanning tunnelling microscopy (STM). Recently, there have been successful attempts to deposit various single-molecule magnets on surfaces using solution-based deposition methods. This can be achieved either by functionalizing the cluster so that it may be grafted onto an Au(111) surface [13] , [14] , [20] , [21] , [22] , [23] , [24] or prefunctionalizing both the substrate and the molecule to encourage the formation of adsorbed layers [25] , [26] , [27] . Deposition in UHV using pulsed laser deposition [28] , matrix-assisted pulsed laser evaporation [29] , a pulsed vacuum spray technique [30] and a local mechanical method [31] has also been demonstrated. However, when applied to the formation of Mn 12 (acetate) 16 films, fragmentation and possible damage to the manganese core [30] , [32] were reported. We used electrospray deposition (ESD) to prepare thin films of Mn 12 (acetate) 16 (structure shown in Fig. 1 ) on an Au(111) surface with coverages ranging from submonolayer to multilayers. It has recently been shown that UHV-ESD and related spray techniques provide a viable method for the transfer of non-volatile/thermally labile species such as dye molecules and polymers from solution onto surfaces held in UHV [33] , [34] , [35] , [36] , [37] , [38] , [39] ; the development and application of this technique is crucial for the deposition of Mn 12 (acetate) 16 . Images of the adsorbed Mn 12 (acetate) 16 are acquired using an STM operating at room temperature under UHV conditions. The operation of the UHV-ESD process and other experimental protocols are described in the Methods section below. 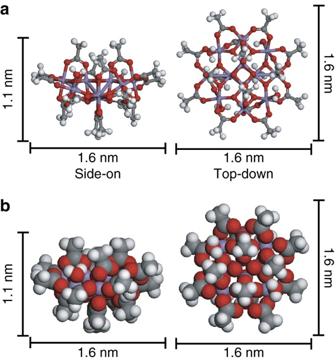Figure 1: Chemical structure of Mn12(acetate)16. (a) Mn12O12(O2CCH3)16(H2O)4(Mn12(acetate)16), (b) structure of Mn12(acetate)16shown as a space-filling model. The dimensions of the molecule are indicated (key: grey, carbon; red, oxygen; lilac, manganese; white hydrogen). Figure 1: Chemical structure of Mn 12 (acetate) 16 . ( a ) Mn 12 O 12 (O 2 CCH 3 ) 16 (H 2 O) 4 (Mn 12 (acetate) 16 ), ( b ) structure of Mn 12 (acetate) 16 shown as a space-filling model. The dimensions of the molecule are indicated (key: grey, carbon; red, oxygen; lilac, manganese; white hydrogen). Full size image 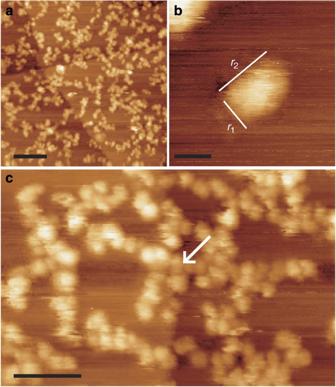Figure 2: STM images of Mn12(acetate)16on Au(111). (a) A large-scale STM image of the Au(111) surface after the UHV-ESD of∼0.35 ml of Mn12(acetate)16(Vsample=+1.80 V,Itunnel=0.03 nA). Filamentary structures are observed to run over the surface and are contiguous at step edges. Scale bar, 20 nm. (b) Closeup STM image of an isolated Mn12(acetate)16molecule (Vsample=+2.00 V,Itunnel=0.03 nA). The molecule displays an elliptical cross-section (r2>r1). Scale bar, 2 nm. (c) STM image showing the internal structure of a molecular aggregate comprised of individual Mn12(acetate)16molecules (Vsample=+2.00 V,Itunnel=0.05 nA). Arrow indicates the position of the structure relative to a step edge. Scale bar, 10 nm. STM of adsorbed Mn 12 (acetate) 16 Figure 2a shows a large area STM image of the surface following the deposition of a submonolayer of Mn 12 (acetate) 16 ( ∼ 0.35 ML (monolayer)). It is immediately clear from this image that the molecules are mobile and diffuse on the surface following adsorption as their positions are nonrandom and they form complex aggregates in which meandering filamentary structures coexist with small disordered clusters. These features are somewhat reminiscent of the filamentary networks reported recently for planar organic molecules [40] , [41] , which have been described as two-dimensional glasses. From a simple consideration of the molecular hard-sphere radius ( Fig. 1b ), it might be expected that the Mn 12 (acetate) 16 molecules would be oriented to maximize the contact area, potentially maximizing the van der Waals interaction with the substrate, giving rise to a circular cross-section in STM images. However, as shown in the STM image of an isolated Mn 12 (acetate) 16 ( Fig. 2b ), the orthogonal dimensions of the molecule, labelled r 1 and r 2 , are not equal, and the molecule is imaged with an ellipsoidal cross-section. The average values of r 1 (short axis) and r 2 (long axis) for isolated molecules have been experimentally measured to be 1.6 ± 0.3 and 2.2 ± 0.4 nm, respectively, with an aspect ratio of 1.4 ± 0.2. The lateral dimensions of Mn 12 (acetate) 16 , as measured by STM, are approximately 30% larger than the hard-sphere radius because of STM tip convolution. The average apparent height of the molecules, 0.45 ± 0.08 nm, is lower than the hard-sphere dimension. This difference is attributed to a lower local density of states associated with the Mn 12 (acetate) 16 , as compared with the metallic Au surface. Figure 2: STM images of Mn 12 (acetate) 16 on Au(111). ( a ) A large-scale STM image of the Au(111) surface after the UHV-ESD of ∼ 0.35 ml of Mn 12 (acetate) 16 ( V sample =+1.80 V, I tunnel =0.03 nA). Filamentary structures are observed to run over the surface and are contiguous at step edges. Scale bar, 20 nm. ( b ) Closeup STM image of an isolated Mn 12 (acetate) 16 molecule ( V sample =+2.00 V, I tunnel =0.03 nA). The molecule displays an elliptical cross-section ( r 2 > r 1 ). Scale bar, 2 nm. ( c ) STM image showing the internal structure of a molecular aggregate comprised of individual Mn 12 (acetate) 16 molecules ( V sample =+2.00 V, I tunnel =0.05 nA). Arrow indicates the position of the structure relative to a step edge. Scale bar, 10 nm. Full size image A striking feature of the molecular assemblies observed using STM is the propensity of the Mn 12 (acetate) 16 molecules to self-assemble into meandering filamentary structures as depicted in Figure 2c . These structures are observed to run over step edges, giving rise to the large-scale surface structure seen in Figure 2a . The formation of these structures is not associated with, and does not follow, the underlying herringbone reconstruction [42] of the Au(111) surface. Interactions between Mn 12 (acetate) 16 and an Au(111) substrate The STM images raise questions as to how the Mn 12 (acetate) 16 molecules are oriented on the surface, and the mechanism that drives the self-assembly of these complex aggregates. Semiempirical molecular dynamics (MD) simulations have been used to obtain information about the energetic states that an individual molecule deposited on to the Au(111) substrate may occupy. 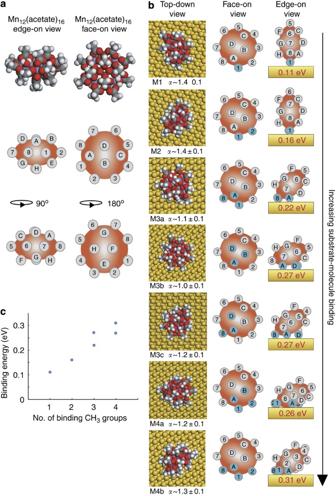Figure 3: Calculated configuration of Mn12(acetate)16on Au(111). (a) Hard-sphere model Mn12(acetate)16and schematic of the molecule with the CH3groups of the molecule's organic shell labelled 1–8 and A–H (grey circles) and the Mn12O12core is represented as a red ellipsoid. (b) The left-hand column shows a top-down view of the states determined to be energy minima of the system (1 Mn12(acetate)16on the Au(111) surface) by the MD quench simulation. The aspect ratio of each state is shown in each case (α). The middle column is a schematic of a face-on view, with the CH3groups in contact with the Au surface highlighted as blue circles. The right-hand column shows an edge-on view rotated by 90° compared with that of side 1, with the CH3groups in contact with the Au surface highlighted as blue circles. The states are shown in the order of increasing bonding energy, M1–M4b. (c) Graph showing the binding energy of the Mn12(acetate)16to the Au surface as a function of the number of CH3groups in contact with the surface. A simple schematic of the molecule, shown in Figure 3a , with the majority of the Mn 12 (acetate) 16 depicted as a red ellipsoid with the protruding CH 3 groups shown as grey circles is used to analyse the MD results. Figure 3: Calculated configuration of Mn 12 (acetate) 16 on Au(111). ( a ) Hard-sphere model Mn 12 (acetate) 16 and schematic of the molecule with the CH 3 groups of the molecule's organic shell labelled 1–8 and A–H (grey circles) and the Mn 12 O 12 core is represented as a red ellipsoid. ( b ) The left-hand column shows a top-down view of the states determined to be energy minima of the system (1 Mn 12 (acetate) 16 on the Au(111) surface) by the MD quench simulation. The aspect ratio of each state is shown in each case ( α ). The middle column is a schematic of a face-on view, with the CH 3 groups in contact with the Au surface highlighted as blue circles. The right-hand column shows an edge-on view rotated by 90° compared with that of side 1, with the CH 3 groups in contact with the Au surface highlighted as blue circles. The states are shown in the order of increasing bonding energy, M1–M4b. ( c ) Graph showing the binding energy of the Mn 12 (acetate) 16 to the Au surface as a function of the number of CH 3 groups in contact with the surface. Full size image There are 16 CH 3 groups in total, eight of which lie around the circumference of the ellipsoid (labelled 1–8), and four on both the top and bottom of the molecule (labelled A–D and E–H, respectively). MD quench simulations were performed on a single Mn 12 (acetate) 16 molecule on the Au(111) substrate. The quench simulation allows geometry optimization calculations to be performed using a variety of starting geometries determined by MD. From the geometry optimized structures, it is possible to identify several distinct local energy minima, each of which may be defined by the orientation of the CH 3 groups relative to the surface. The left-hand column of Figure 3c shows a top-down view of the geometry-optimized energy minima with the values for their aspect ratios. The middle column shows schematic representations of the molecule in which the CH 3 groups in contact with the Au(111) surface are highlighted for each orientation. The edge-on view in the right-hand column shows how the molecules are oriented relative to the surface with the CH 3 groups in contact with the surface highlighted in blue. States M1 and M2 (identified in Fig. 3 ) are energy minima in which the molecule is positioned perpendicular to the gold surface, whereas in state M3b, the molecule lies almost flat on the surface. The lowest energy state (state M4b) shows that the molecule is canted so that four CH 3 groups are in contact with the surface. The energies of the states have been plotted as a function of the number of CH 3 groups in contact with the surface ( Fig. 3c ). The graph shows a linear trend, which demonstrates that the binding energy of the molecule to the surface, and hence the molecular orientation, is determined by the number of CH 3 groups in contact with the Au(111) surface. State M4b has the greatest binding energy (0.31 ± 0.02 eV), and the geometry of this state gives a top-down aspect ratio of 1.3 ± 0.1, which is in agreement with the value obtained from the STM images. Interactions between adsorbed Mn 12 (acetate) 16 molecules The simulations also provide insight into the formation of the complex aggregates of Mn 12 (acetate) 16 molecules on the Au(111) surface. A similar approach to that described above is taken with a quench simulation being performed to determine the energy minima for a system containing two Mn 12 (acetate) 16 molecules absorbed on Au(111). 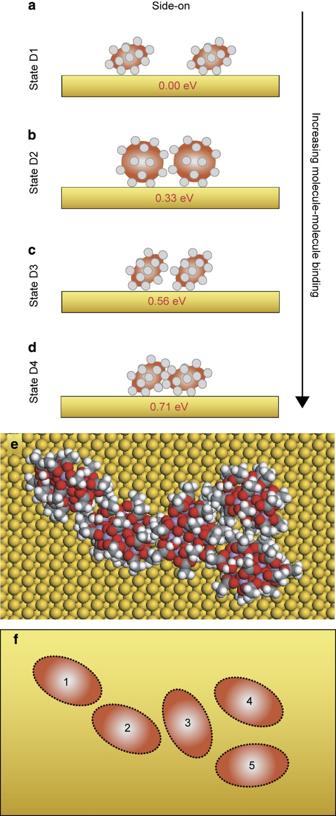Figure 4: Calculated configurations of Mn12(acetate)16pairs. (a–d) Schematics showing the energy minima of the molecule–molecule interaction between two Mn12(acetate)16molecules. (e) Final structure from an MD simulation of five Mn12(acetate)16molecules on an Au(111) surface showing the formation of a meandering chain-like structure. (f) Schematic showing the positions of the five Mn12(acetate)16molecules at the end of the MD simulation. Figure 4a–d shows the geometry of the four local energy minima states for two molecules. For each state, the binding energy between the two molecules has been calculated, with state D1 defined as a non-bonding configuration with the molecules not in contact. State D2 shows an edge-to-edge configuration, whereas states D3 and D4 show face-to-face configurations in which the surface area between the two interacting molecules is maximized (the substrate interaction is included in the calculation but is approximately equal for all pair configurations and has been subtracted from the quoted values, which thus correspond to intermolecular interactions—see Supplementary Information for more details). Importantly, the binding energy of state D4 is considerably greater than that of state D3 because of the interdigitation of the methyl groups. Figure 4: Calculated configurations of Mn 12 (acetate) 16 pairs. ( a – d ) Schematics showing the energy minima of the molecule–molecule interaction between two Mn 12 (acetate) 16 molecules. ( e ) Final structure from an MD simulation of five Mn 12 (acetate) 16 molecules on an Au(111) surface showing the formation of a meandering chain-like structure. ( f ) Schematic showing the positions of the five Mn 12 (acetate) 16 molecules at the end of the MD simulation. Full size image The determination of these states allows us to identify the anisotropy in the binding energy between pairs of molecules, which manifests itself in the formation of filamentary structures. Interestingly, the two molecules in the most strongly bound pair arrangement (D4) adopt inequivalent surface configurations with, for example, a difference in tilt angle of ∼ 15°, as illustrated schematically in Figure 4 . One consequence of this is that a given molecule cannot maximize its pairwise intermolecular interactions with more than one of its nearest neighbours. We may therefore expect a competition and interdependency between interactions with multiple several nearest neighbours. Overall, we may expect the molecular shape asymmetry to lead to a complex intermolecular potential that promotes an overall anisotropy through the face-to-face configuration but has several local minima leading to large multiplicity of quasi-degenerate configurations for an arrangement of many molecules. From this perspective, the Mn 12 (acetate) 16 morphology may be seen as analogous to the networks described recently as glasses [40] , [41] . Figure 4e shows the results of an MD simulation in which the positions of five Mn 12 (acetate) 16 molecules on an Au(111) substrate have evolved over time. The resultant structure is a meandering quasi-1D arrangement of molecules similar to those observed in STM images. Figure 4f shows a schematic of the final configuration, with the molecules labelled 1 and 2 clearly adopting the state D2 type of bonding configuration, whereas molecules 3, 4 and 5 adopt conformations similar to states D3 and D4. It is important to note that the magnetic properties of Mn 12 (acetate) 16 are unlikely to be the driving force behind the formation of the observed structures. The MD simulations do not include any information about the magnetic interactions, and the blocking temperature of Mn 12 (acetate) 16 , that is, the temperature at which the magnetic spin will not relax back to its ground state, is 4K [43] , so that magnetic ordering is not expected at room temperature. NEXAFS studies of the adsorbed Mn 12 (acetate) 16 The stability of Mn 12 (acetate) 16 against this deposition process is confirmed by near-edge X-ray absorption fine-structure (NEXAFS) measurements acquired at beamline D1011 of the MAX-Lab synchrotron radiation facility. 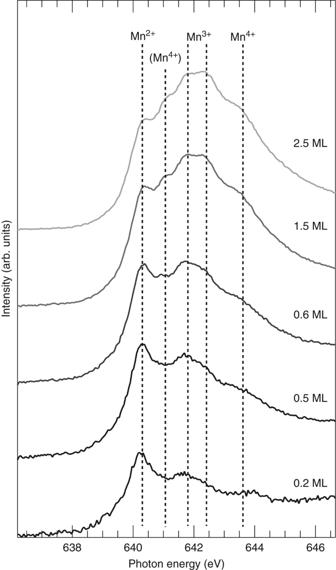Figure 5: NEXAFS spectra measured at the Mn 2padsorption edge (Mn L-edge). Spectra were acquired for a range of coverages (0.2–2.5 ML (monolayer)). Photon energy was calibrated by measuring the energy separation of the Au 4fcore-level photoemission peaks excited by first- and second-order X-rays. The positions of the peaks corresponding to the presence of Mn2+, Mn3+and Mn4+are labelled. Figure 5 shows NEXAFS spectra taken at the Mn2 p adsorption edge for coverages between 0.2 and 2.5 ML from which the oxidation state of the manganese atoms in the core of the molecule may be identified. Figure 5: NEXAFS spectra measured at the Mn 2 p adsorption edge (Mn L-edge). Spectra were acquired for a range of coverages (0.2–2.5 ML (monolayer)). Photon energy was calibrated by measuring the energy separation of the Au 4 f core-level photoemission peaks excited by first- and second-order X-rays. The positions of the peaks corresponding to the presence of Mn 2+ , Mn 3+ and Mn 4+ are labelled. Full size image For multilayer coverages, the NEXAFS spectra are consistent with a mixture of Mn 3+ and Mn 4+ oxidation states, similar to that previously observed [44] for the undamaged Mn 12 (acetate) 16 molecule. However, for submonolayer coverages (0.2, 0.5 and 0.6 ML), the spectra observed are consistent with that of a sample consisting predominantly of the Mn 2+ oxidation state. This analysis is based on a comparison with NEXAFS data acquired for a reference sample of MnO [44] , [45] , which contains only the Mn 2+ oxidation state and is characterized by a large peak in the NEXAFS spectra at ∼ 640 eV (labelled as Mn 2+ in Fig. 5 ) [44] . From this comparison, we may assert that for submonolayer coverages of Mn 12 (acetate) 16 deposited by UHV-ESD, the majority oxidation state for the Mn atoms is 2+. In accordance with previous studies [46] , we observe the growth of a peak over several hours corresponding to the Mn 2+ oxidation state. This time-dependent feature is attributed to beam damage and was observed for all coverages. However, we stress that our observation of Mn 2+ oxidation for submonolayer coverage is not due to beam damage and all spectra shown are acquired immediately after the initial exposure to the beam, before beam damage occurs. Indeed, the features labelled Mn 3+ ( ∼ 642.0 eV) and Mn 4+ (643.5 eV) in Figure 5 grow dramatically as the coverage is increased, confirming that the reduction is a surface-mediated effect. The mechanism for reduction may be due to direct charge transfer from the surface or may arise from internal changes to the bonding of the Mn 12 O 12 core, possibly because of surface-induced modification or even loss of the attached H 2 O or acetate ligands. A simple charge transfer from the surface would likely be associated with a strong surface-core bonding, which is unlikely to be compatible with the observed diffusivity of the Mn 12 (acetate) 16 ; we therefore suggest that the second possibility is more likely. Modification of the shell ligands would naturally lead to corrections to our simple numerical model, but the overall hypothesis that anisotropic interactions result from shape asymmetry is expected to remain valid. Overall, the expected oxidation states for an intact molecule are observed for multilayer coverage, confirming that the chemical properties of Mn 12 (acetate) 16 are unaffected by the UHV-ESD process. Mn 12 (acetate) 16 adsorbed on a supramolecular network The adsorbed Mn 12 (acetate) 16 may be induced to form structures with different order when deposited on a surface on which a hydrogen-bonded nanoporous network has been prepared. We have previously shown that nanoporous supramolecular templates can be formed on the Au(111) surface by combining the organic building blocks PTCDI (3,4,9,10-perylene tetracarboxylic diimide) and melamine (1,3,5-triazine-2,4,6-triamine) [33] , [47] , [48] . The pores within such a network have been shown to function as nanoscale traps for diffusing molecules [2] , [49] , [50] , [51] , [52] , [53] , including, for low coverage, molecular species deposited by UHV-ESD. 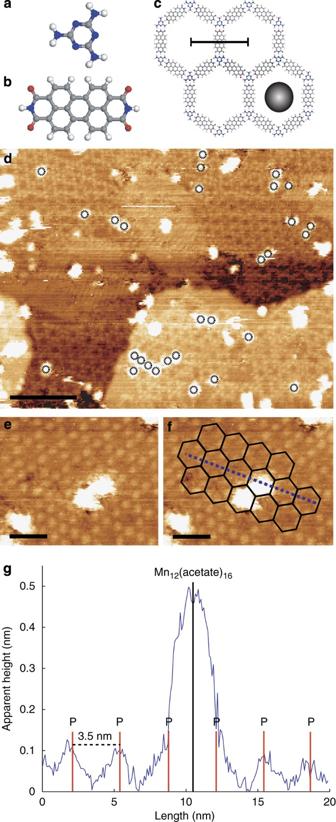Figure 6: Mn12(acetate)16adsorbed on a supramolecular network. Chemical structures of (a) melamine (1,3,5-triazine-2,4,6-triamine) and (b) PTCDI (3,4,9,10-perylene tetracarboxylic diimide). (c) Structure of the self-assembled hexagonal network formed by the hydrogen bonding interaction between melamine and PTCDI (key: grey, carbon; red, oxygen; blue, nitrogen; white, hydrogen). The grey circle represents the size of an Mn12(acetate)16relative to the dimensions of the network (the highlighted pore separation is 3.5 nm). From geometric considerations, one Mn12(acetate)16may be trapped within each pore. (d) STM image of the Au(111) surface that has been prepatterned with a melamine/PTCDI network before the UHV-ESD of Mn12(acetate)16(Vsample=+1.80 V,Itunnel=0.03 nA). Dashed black circles highlight Mn12(acetate)16trapped within a network pore. Scale bar, 20 nm. (e) Closeup STM image showing two Mn12(acetate)16molecules trapped within neighbouring network pores (Vsample=+1.80 V,Itunnel=0.03 nA). Scale bar, 5 nm. (f) STM image from (e), with an overlay highlighting the position of the hexagonal network. Scale bar, 5 nm. (g) Line profile taken over a region of network containing one trapped Mn12(acetate)16. The path of the line profile is shown in (f) and the positions of PTCDI molecules are labelled P. The location of the trapped Mn12(acetate)16in the centre of the pore is marked. Figure 6a–c shows the structure of melamine, PTCDI and the structure of the hexagonal network, respectively. From a comparison of the dimensions of the hexagonal pores (width ∼ 2.5 nm) and the Mn 12 (acetate) 16 , it is expected that each pore would have the capacity for one molecule. Figure 6d shows an Au(111) substrate that has been prepatterned with a melamine/PTCDI hexagonal network and been exposed to a deposition of 0.05 monolayers of Mn 12 (acetate) 16 by UHV-ESD. The positions of Mn 12 (acetate) 16 molecules held within a pore of this host/guest architecture are highlighted (in addition, some non-highlighted Mn 12 (acetate) 16 molecules are adsorbed at other sites on the surface), and it can be seen that the resultant structure demonstrates a trapping of the molecules within the pores. This result shows that hydrogen-bonded supramolecular networks have the potential to trap Mn 12 (acetate) 16 deposited by UHV-ESD and locally inhibit the formation of filaments, such as those discussed above, or other molecular aggregates. Figure 6e,f show closeup STM images of the hexagonal network containing two trapped Mn 12 (acetate) 16 molecules, with the overlay in Figure 6f highlighting the positions of the network pores. A line profile is shown in Figure 6g (the path of the line profile is depicted in Fig. 6f ) from which the periodicity of the hexagonal network and the position of the trapped Mn 12 (acetate) 16 may be determined. Interestingly, there is an indication in this image that the occupancy of neighbouring host sites is slightly correlated. A similar effect for the capture of C 60 dimers was reported previously by Staniec et al . [48] and attributed to a kinetic effect, although for the Mn 12 (acetate) 16 , an energetic origin is also possible. Figure 6: Mn 12 (acetate) 16 adsorbed on a supramolecular network. Chemical structures of ( a ) melamine (1,3,5-triazine-2,4,6-triamine) and ( b ) PTCDI (3,4,9,10-perylene tetracarboxylic diimide). ( c ) Structure of the self-assembled hexagonal network formed by the hydrogen bonding interaction between melamine and PTCDI (key: grey, carbon; red, oxygen; blue, nitrogen; white, hydrogen). The grey circle represents the size of an Mn 12 (acetate) 16 relative to the dimensions of the network (the highlighted pore separation is 3.5 nm). From geometric considerations, one Mn 12 (acetate) 16 may be trapped within each pore. ( d ) STM image of the Au(111) surface that has been prepatterned with a melamine/PTCDI network before the UHV-ESD of Mn 12 (acetate) 16 ( V sample =+1.80 V, I tunnel =0.03 nA). Dashed black circles highlight Mn 12 (acetate) 16 trapped within a network pore. Scale bar, 20 nm. ( e ) Closeup STM image showing two Mn 12 (acetate) 16 molecules trapped within neighbouring network pores ( V sample =+1.80 V, I tunnel =0.03 nA). Scale bar, 5 nm. ( f ) STM image from ( e ), with an overlay highlighting the position of the hexagonal network. Scale bar, 5 nm. ( g ) Line profile taken over a region of network containing one trapped Mn 12 (acetate) 16 . The path of the line profile is shown in ( f ) and the positions of PTCDI molecules are labelled P. The location of the trapped Mn 12 (acetate) 16 in the centre of the pore is marked. Full size image Our study demonstrates that molecules such as the single-molecule magnet Mn 12 (acetate) 16 can form complex aggregates when adsorbed at submonolayer coverages on an Au(111) surface. The growth of the filamentary aggregates is due to an anisotropic intermolecular interaction. In this case, the anisotropy is a direct consequence of the van der Waals interactions among the acetate ligands that are asymmetrically arranged around the Mn 12 core, and does not arise from chemically specific interactions. The interlocking of these groups may be considered as a three-dimensional analogue of the alkyl chain interdigitation as observed for planar molecules [54] . Our results show that the growth of materials from the vapour deposition of large molecules, which lack a high degree of symmetry, can give rise to highly complex structures, and that such aggregated structures can be modelled using MD simulations. We also show that the approach of supramolecular templating can influence the lateral organization of large three-dimensional molecular nanoparticles, in addition to small molecules, as has previously been considered. We anticipate that the combination of UHV-ESD and surface adsorption will find wide relevance for the controlled formation of nanostructured surfaces based not only on Mn 12 (acetate) 16 , as considered here, but also with many other large molecules. Sample preparation and STM imaging Deposition of Mn 12 (acetate) 16 and subsequent characterization by STM were carried out using a UHV system with a base pressure of ∼ 5×10 −11 Torr; separate chambers were used for deposition and characterization. A 4×8 mm gold on mica substrate (thickness of 1500 Å; supplied commercially by Agilent) was loaded into the UHV system. The sample was cleaned by Ar ion sputtering (6×10 −6 Torr, 0.7 keV, ∼ 2 μA) and subsequent annealing ( ∼ 500 °C). Images of the surface were acquired using a scanning tunnelling microscope, housed within the UHV system, using electrochemically etched tungsten tips, and operating in constant current mode at room temperature. Images of the surface taken after the sputter–anneal cycle show the characteristic (22×√3) herringbone reconstruction of the Au(111) surface [42] . UHV-ESD Using UHV-ESD, Mn 12 (acetate) 16 was transferred from a solution of methanol onto the Au(111) substrate. The UHV-ESD experimental setup has been described in detail previously [33] , [34] . To summarize, a solution containing the molecules to be deposited is passed through a stainless steel emitter held at ∼ 2 kV at a typical flow rate of 1 μl min −1 . This leads to the formation of a spray at atmospheric pressure outside the UHV system. The spray enters the UHV system through an aperture, passes through a series of differentially pumped chambers and impinges on the sample situated within a preparation chamber having a base pressure of 5×10 −11 Torr. The pressure in the sample preparation chamber while open to the differential pumping system, but in the absence of spray, is ∼ 2×10 −8 Torr. During ESD, the pressure rises to ∼ 4×10 −8 Torr, with the additional pressure being solely due to the presence of solvent molecules within the preparation chamber (ascertained by residual gas analysis). Details of synchrotron-based experiments NEXAFS experiments were conducted at the bending magnet beamline D1011 at Max II, MAX-lab in Lund. The D1011 end station is equipped with a SCIENTA SES200 electron analyser, with the base pressure within the analysis and preparation chambers being 2×10 −10 and 4×10 −10 Torr, respectively. For the NEXAFS experiments, the sample was oriented at normal emission relative to the analyser. The sample used was a single crystal Au(111) substrate with a 10 mm diameter (2.5 mm thickness) purchased from Metal Crystals and Oxides. A loop of tungsten wire was passed through the crystal to mount it and provide resistive heating, with a thermocouple wire being attached within a small cavity to monitor the temperature. The sample was cleaned using cycles of argon sputtering (1 keV) and annealing (600 °C) until it showed a negligible C1 s core-level signal. C1 s core-level spectra were measured using h ν=340 eV. Mn NEXAFS data were recorded at the Mn 2p adsorption edge (Mn L-edge) with the emitted electrons collected by a partial yield detector, with a retardation potential of 100 V. The photon energy was calibrated by taking the energy separation of the Au 4 f core-level photoemission peaks excited by X-rays in first and second order. Coverages were calibrated by comparing the attenuation of the Au4 f substrate peak with that of the clean Au(111) sample, with the mean free path through the Mn 12 (acetate) 16 calculated using the Seah and Dench method [55] . Details of the molecular mechanics simulations Molecular mechanics simulations were performed using the Forcite package within Materials Studio 4.3 (Accelrys). Quench calculations were used to obtain the energy minima for a single Mn 12 (acetate) 16 molecule on the Au(111) surface. In these quench calculations, an MD simulation is performed, and at periodic intervals the geometry from the MD simulation is used as the starting point for a geometry optimization calculation, allowing a range of starting geometries to be sampled. The simulations of a single Mn 12 (acetate) 16 molecule on the Au(111) surface were performed using periodic boundary conditions (cell dimensions A =43.2569 Å, B =43.2569 Å, C =54.7092 Å, α =90°, β =90°, γ =120°), with the molecule being placed at the centre of the cell on top of a 3-ML slab of the Au(111) surface, and with the Au atoms of the substrate being constrained throughout the calculations. The formal charges for Mn were set so that the four central atoms had a charge of +4 and the eight outer atoms had a charge of +3. The charge equilibration (QEq) method was used to distribute the charge across the molecule [56] . The universal force field was used to describe the atoms within the molecule, and the atoms within the Au(111) surface, with no changes being made to the automatically assigned force field typings [57] . The calculation parameters are presented in Supplementary Table S1 . After the quench calculation was performed, the binding energy (BE) of Mn 12 (acetate) 16 to the Au(111) surface was calculated. A graph showing the different BEs obtained for structures optimized from different starting geometries, obtained from the quench simulation, is shown in Supplementary Figure S1 . From these energies, it is possible to characterize energetic states in terms of the geometric arrangement of the molecule, relative to the surface (state geometries are shown in Supplementary Fig. S2 , with the BEs summarized in Supplementary Table S2 ). Quench simulations were carried out for two Mn 12 (acetate) 16 molecules situated on an Au(111) surface as described above. The BE between the two molecules has been calculated at each quench step and is shown in Supplementary Figure S3 . As with the case of an isolated Mn 12 (acetate) 16 molecule adsorbed on the Au(111) surface, we are able to identify discrete states for the interaction between two such molecules. The energies corresponding to the discrete states defined in Figure 4 are presented in Supplementary Table S3 . An MD calculation to simulate the motion of five molecules on the Au(111) surface was performed using the parameters in Supplementary Table S4 . The simulations were performed using periodic boundary conditions (cell dimensions A =86.5138 Å, B =86.5138 Å, C =54.7092 Å, α =90°, β =90°, γ =120°), with the molecules being placed in the cell on top of a 3-ML slab of the Au(111) surface, and with the Au atoms of the substrate being constrained throughout the calculations. Supplementary Figure S4 shows the initial and final frames of the simulation. How to cite this article: Saywell, A. et al . Self-assembled aggregates formed by single-molecule magnets on a gold surface. Nat. Commun. 1:75 doi: 10.1038/ncomms1075 (2010).